Identity of endogenous NMDAR glycine site agonist in amygdala is determined by synaptic activity level Mechanisms of N -methyl- D- aspartate receptor-dependent synaptic plasticity contribute to the acquisition and retention of conditioned fear memory. However, synaptic rules which may determine the extent of N -methyl- D- aspartate receptor activation in the amygdala, a key structure implicated in fear learning, remain unknown. Here we show that the identity of the N -methyl- D- aspartate receptor glycine site agonist at synapses in the lateral nucleus of the amygdala may depend on the level of synaptic activation. Tonic activation of N -methyl- D- aspartate receptors at synapses in the amygdala under low activity conditions is supported by ambient D -serine, whereas glycine may be released from astrocytes in response to afferent impulses. The release of glycine may decode the increases in afferent activity levels into enhanced N -methyl- D- aspartate receptor-mediated synaptic events, serving an essential function in the induction of N -methyl- D- aspartate receptor-dependent long-term potentiation in fear conditioning pathways. Activation of N -methyl- D- aspartate receptors (NMDARs) by glutamate in the brain defines many crucial biological processes, including learning, memory and developmental plasticity [1] , [2] . Unlike other neurotransmitter receptors, activation of NMDARs requires simultaneous occupation of two different binding sites by glutamate and the glycine site agonist, respectively [3] , [4] , [5] . Previous experimental findings provided evidence for the role of either glycine [6] , [7] , [8] or D- serine [9] , [10] , [11] , [12] as the endogenous NMDAR glycine site agonist at central synapses. Glycine may be accumulated by astrocytes, expressing the glycine transporter GlyT1, and could be released by them through the mechanisms of reverse transport in response to the local increases in the intra-astrocyte Na + concentration, possibly due to activation of astrocytic α-amino-3-hydroxy-5-methyl-4-isoxazolepropionic acid (AMPA) receptors [13] , [14] , [15] . D- serine can also be released from astrocytes via mechanisms implicating Ca 2+ and SNARE-dependent exocytosis [10] , [12] , [16] (but see Agulhon et al . [17] ) or from neurons [18] via a nonvesicular release mechanism [19] . Whereas the results of earlier experiments suggested that tonically present glycine could saturate the NMDA receptor glycine site [20] , it has been shown in subsequent studies that glycine transporters decrease the concentration of glycine at synaptic sites below the saturation level [6] , [7] , [21] . Consistent with the latter finding, it has been demonstrated that the degree of NMDAR activation could be regulated through the changes in the glycine site occupancy [8] , [22] . The lack of the glycine site saturation, however, is not universal, as the glycine site was shown to be saturated by endogenous coagonist at the cerebellar mossy fibres to granule cell synapses [23] . This indicates that the level of the glycine site occupancy by the coagonist under baseline conditions might reflect characteristics of particular synaptic connections. Notably, there is evidence that the NMDAR glycine site might be unsaturated at central synapses in vivo [24] , [25] , indicating that the results on modulation of the NMDARs in acute brain slices could be extrapolated to the certain degree to the in vivo situation. Little is known, however, about the most fundamental aspects of NMDAR function in the amygdala, a key brain structure in fear-related behaviours [26] , [27] . This is an important issue as the acquisition of conditioned fear, resulting from a formation of the association between conditioned and unconditioned stimuli (CS and US, respectively), is NMDAR dependent [28] , [29] , [30] and implicates the mechanisms of NMDA receptor-dependent plasticity in the CS pathways [31] , [32] , [33] , [34] , [35] , [36] , [37] . Surprisingly, the identity of the endogenous NMDA receptor glycine site agonist in amygdala remains undetermined. Another fundamental question, which has not been addressed in any region of the brain, is whether the identity of the coagonist is unchanged while signals propagate within the neuronal network or it might be related to the afferent activity patterns. We addressed these questions by studying the mechanisms of NMDAR activation under different degrees of afferent activity. We found that the identity of the NMDAR glycine site agonist at synapses in the lateral nucleus of the amygdala (LA), glycine or D- serine, is determined by the level of synaptic activity, affecting the inducibility of long-term potentiation (LTP) in the auditory CS pathways. D- serine is glycine site agonist under low activity levels To identify the endogenous NMDAR coagonist at synapses in the LA, we recorded either spontaneous excitatory postsynaptic currents (sEPSCs) or evoked EPSCs in acute brain slices treated with either D- amino acid oxidase (DAAO) or glycine oxidase (GO), enzymes catabolizing endogenous D- serine or glycine, respectively [11] . We focused in our studies on LA synapses [26] , [27] because NMDAR-dependent LTP in cortical and thalamic inputs to the LA was linked previously to the acquisition of fear memory [32] , [33] , [34] . Importantly, we found in control slices that, similar to hippocampal synapses [7] , [8] , the glycine site of the NMDAR in LA neurons is not saturated by the ambient endogenous coagonist, which, nevertheless, supports tonic activation of NMDARs under baseline conditions ( Supplementary Fig. S1 ). Consistent with the role of D- serine as an endogenous coagonist of the NMDAR glycine site, the amplitude of the NMDAR-mediated component of sEPSCs, recorded at a holding potential of +40 mV ( Supplementary Fig. S1 ), was decreased after incubation of slices in the external solution containing DAAO ( Fig. 1a ). Subsequent application of D- serine (10 μM) reversed the effects of DAAO on NMDAR sEPSCs, potentiating them to the same degree as in untreated slices. Thus, the observed decreases in the amplitude of the NMDAR sEPSCs were not due to direct damage to the NMDARs by the enzymatic treatment. The size of the NMDAR sEPSCs remained unchanged, however, in slices treated with GO ( Fig. 1c ). 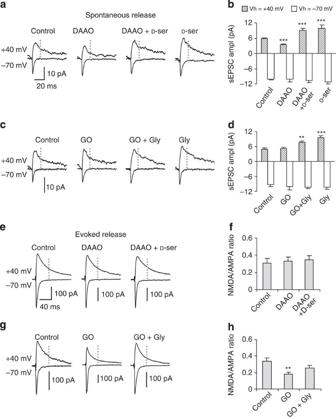Figure 1:D-serine supports tonic NMDAR activation and glycine serves as the glycine site agonist during afferent stimulation. (a) Averaged sEPSCs (50–100 events) recorded from LA neurons at −70 mV or +40 mV under control conditions, following treatment of slices with DAAO (45 min; 0.17 unit ml−1), and after addition ofD-serine (10 μM) to treated or control slices. NMDAR-mediated component was measured at +40 mV (dashed lines). (b) Summary of experiments as ina. Control,n=9 neurons; DAAO,n=10; DAAO+D-serine,n=8;D-serine alone,n=10. NMDAR current was decreased following the treatment (t-test, ***P<0.001 versus control). NMDAR current was potentiated in the DAAO+D-serine or controlD-serine groups (***P<0.001).P=0.6 between DAAO+D-serine andD-serine only groups. AMPAR EPSCs at −70 mV remained unchanged. (c) Slices were treated with GO (45 min; 0.04 unit ml−1) and glycine (10 μM) was applied after the treatment or under control conditions. (d) Summary of experiments as inc. Control,n=7 neurons; GO,n=14; GO+glycine,n=9; glycine alone,n=5.P=0.62 for GO versus control, **P=0.004 for control versus GO+glycine,t-test.P=0.06 between GO+glycine and glycine only groups. ***P<0.001 for glycine alone versus control. (e) Averaged traces (15 responses) of evoked thalamo-LA EPSCs recorded at −70 mV and +40 mV under three conditions: control, after DAAO treatment and after addition ofD-serine (10 μM) to DAAO-treated slices. (f) Summary plot of the NMDA/AMPA amplitude ratios for experiments as ine. Control,n=10 neurons; DAAO,n=11; DAAO+D-serine,n=6.P=0.8 for control versus DAAO group;P=0.55 for DAAO versus DAAO+D-serine,t-test. (g) Slices were treated with GO. (h) Summary of experiments as ing. NMDA/AMPA ratio: control,n=13 neurons; GO,n=12; GO+glycine,n=6. **P=0.002 for control versus GO group,t-test.P=0.16 for control versus GO+glycine. Error bars are s.e.m. Figure 1: D- serine supports tonic NMDAR activation and glycine serves as the glycine site agonist during afferent stimulation. ( a ) Averaged sEPSCs (50–100 events) recorded from LA neurons at −70 mV or +40 mV under control conditions, following treatment of slices with DAAO (45 min; 0.17 unit ml −1 ), and after addition of D- serine (10 μM) to treated or control slices. NMDAR-mediated component was measured at +40 mV (dashed lines). ( b ) Summary of experiments as in a . Control, n =9 neurons; DAAO, n =10; DAAO+ D- serine, n =8; D- serine alone, n =10. NMDAR current was decreased following the treatment ( t -test, *** P <0.001 versus control). NMDAR current was potentiated in the DAAO+ D- serine or control D- serine groups (*** P <0.001). P =0.6 between DAAO+ D- serine and D- serine only groups. AMPAR EPSCs at −70 mV remained unchanged. ( c ) Slices were treated with GO (45 min; 0.04 unit ml −1 ) and glycine (10 μM) was applied after the treatment or under control conditions. ( d ) Summary of experiments as in c . Control, n =7 neurons; GO, n =14; GO+glycine, n =9; glycine alone, n =5. P =0.62 for GO versus control, ** P =0.004 for control versus GO+glycine, t -test. P =0.06 between GO+glycine and glycine only groups. *** P <0.001 for glycine alone versus control. ( e ) Averaged traces (15 responses) of evoked thalamo-LA EPSCs recorded at −70 mV and +40 mV under three conditions: control, after DAAO treatment and after addition of D- serine (10 μM) to DAAO-treated slices. ( f ) Summary plot of the NMDA/AMPA amplitude ratios for experiments as in e . Control, n =10 neurons; DAAO, n =11; DAAO+ D- serine, n =6. P =0.8 for control versus DAAO group; P =0.55 for DAAO versus DAAO+ D- serine, t -test. ( g ) Slices were treated with GO. ( h ) Summary of experiments as in g . NMDA/AMPA ratio: control, n =13 neurons; GO, n =12; GO+glycine, n =6. ** P =0.002 for control versus GO group, t -test. P =0.16 for control versus GO+glycine. Error bars are s.e.m. Full size image Detailed characterization of the functional activity of DAAO or GO under experimental conditions, which were very similar to those in our work, has been provided in previous studies [11] , [38] . To demonstrate the specificity of the effects of DAAO or GO under our experimental conditions, we evaluated the effects of enzymatic treatments on D- serine and glycine concentrations by performing high-performance liquid chromatography (HPLC) analysis. In these experiments, D- serine and glycine were detected in the external solution which was bathing slices for 45 min. We found that concentrations of D- serine or glycine decreased significantly in slices treated for 45 min with DAAO (0.17 U ml −1 ) or GO (0.04 U ml −1 ), respectively ( Supplementary Fig. S2 ). The effects of treatments on D- serine or glycine were enzyme specific, as DAAO degraded D- serine but not glycine, whereas GO reduced glycine concentration but had no effect on D- serine. These results provide evidence that enzymes were, in fact, degrading D- serine or glycine in our experiments. The decreases in the amplitude of spontaneous miniature NMDAR-mediated currents (mEPSCs) were also observed when DAAO was applied in the presence of the Na + channel blocker tetrodotoxin (TTX, 1 μM), suppressing spontaneous network activity ( Supplementary Fig. S3 ). It indicates that ambient D- serine, but not glycine, maintains synaptic activation of NMDARs in LA neurons under resting or low activity conditions. Synaptic activity defines identity of glycine site agonist Next, we recorded evoked synaptic currents in thalamic projections to the LA [39] , induced repetitively by single presynaptic stimuli at a stimulation frequency of 0.1 Hz delivered to the internal capsule in the brain slices [36] . The NMDAR-mediated synaptic current component was measured 40 ms after the peak of AMPAR EPSCs (assayed at −70 mV) at +40 mV, thus minimizing a contamination by the AMPAR-mediated synaptic current [40] ( Supplementary Fig. S4 ). Unexpectedly, the NMDA/AMPA amplitude ratio of the averaged evoked EPSCs, which provides an internally controlled measure of changes in the size of the NMDAR-mediated synaptic responses, was unaffected by the treatment with DAAO ( Fig. 1e ). On the other hand, the averaged NMDA/AMPA amplitude ratio was decreased dramatically following the treatment of slices with GO ( Fig. 1g ). The effect of GO was specific to its enzymatic action, because it was not observed when GO activity was inhibited with glycolate [41] (2 mM; Supplementary Fig. S5 ). This suggests that glycine, but not D- serine, is the NMDA receptor glycine site agonist in the LA during continuous synaptic activation by the afferent pulses. A potential problem with the experiments involving the treatment of slices with enzymes, DAAO or GO, is that it could be associated with generation of reaction products that might affect receptor properties (for example, H 2 O 2 ). To address this issue, we tested the effects of DAAO or GO on spontaneous and evoked EPSCs in the presence of catalase (45 min; 100 U ml −1 ; Auerbach et al . [42] ) in external solution. We found that the effects of enzymes were identical to their effects without catalase treatment, with DAAO affecting NMDAR-mediated component of sEPSCs and GO affecting evoked NMDAR EPSCs only ( Supplementary Fig. S6 ). In concord with these findings, the NMDAR-mediated component of sEPSCs was diminished in slices from genetically modified mice that constitutively lack serine racemase [43] , the enzyme that synthesizes endogenous D- serine [44] ( Fig. 2a ). The lack of D- serine, however, had no effect on the NMDA/AMPA amplitude ratio of evoked EPSCs recorded in slices from SR −/− mice ( Fig. 2c ), thus arguing further against a role of D- serine in activity-dependent activation of NMDA receptors in the LA. Confirming specificity of the mutation effect, we found that the treatment of slices from SR −/− mice with DAAO did not affect the NMDAR-mediated component of sEPSCs ( Supplementary Fig. S7 ). Taken together, these findings demonstrate that both D- serine or glycine may serve as endogenous NMDAR coagonists at synapses in the LA in correspondence with the level of synaptic activity. Thus, ambient D- serine appears to provide tonic activation of NMDARs, while glycine serves as a phasic modulator which may be released upon synaptic stimulation. 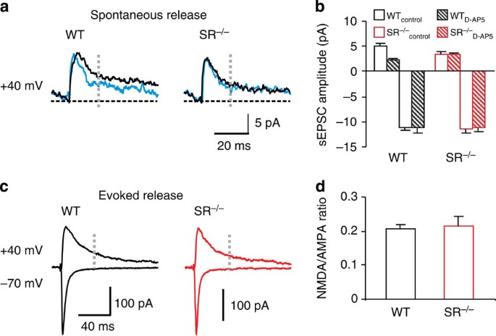Figure 2: NMDAR-mediated component of sEPSCs is diminished in slices from SR−/−mice. (a) Traces of sEPSCs recorded in LA neurons from control (WT) or SR−/−mice at +40 mV under control conditions (black traces) or in the presence of D-AP5 (50 μM, blue traces). Traces are averages of 100–150 sEPSCs at each holding potential. (b) Summary plot showing the peak amplitude of AMPAR sEPSC at −70 mV and the NMDAR-mediated component of the sEPSC at +40 mV (dashed lines) in slices from control (n=9 neurons from three mice) and SR−/−mice (n=10 neurons from four mice). The amplitude of the NMDAR component of the sEPSC was smaller in slices from SR−/−mice (P<0.01 between groups,t-test). The effect of D-AP5 was highly significant in slices from control mice (P<0.01) but not in slices from SR−/−mice (P=0.09). (c) Averaged traces (15 responses) of evoked thalamo-LA EPSCs recorded in LA neuron at −70 mV (bottom) and +40 mV (top) in slices from control or SR−/−mice. (d) Summary of experiments as incshowing the NMDA/AMPA amplitude ratios in slices from control (n=10 neurons from six mice) and SR−/−mice (n=20 neurons from five mice; no significant difference between groups,P=0.9,t-test). Results are shown as means±s.e.m. Figure 2: NMDAR-mediated component of sEPSCs is diminished in slices from SR −/− mice. ( a ) Traces of sEPSCs recorded in LA neurons from control (WT) or SR −/− mice at +40 mV under control conditions (black traces) or in the presence of D-AP5 (50 μM, blue traces). Traces are averages of 100–150 sEPSCs at each holding potential. ( b ) Summary plot showing the peak amplitude of AMPAR sEPSC at −70 mV and the NMDAR-mediated component of the sEPSC at +40 mV (dashed lines) in slices from control ( n =9 neurons from three mice) and SR −/− mice ( n =10 neurons from four mice). The amplitude of the NMDAR component of the sEPSC was smaller in slices from SR −/− mice ( P <0.01 between groups, t -test). The effect of D-AP5 was highly significant in slices from control mice ( P <0.01) but not in slices from SR −/− mice ( P =0.09). ( c ) Averaged traces (15 responses) of evoked thalamo-LA EPSCs recorded in LA neuron at −70 mV (bottom) and +40 mV (top) in slices from control or SR −/− mice. ( d ) Summary of experiments as in c showing the NMDA/AMPA amplitude ratios in slices from control ( n =10 neurons from six mice) and SR −/− mice ( n =20 neurons from five mice; no significant difference between groups, P =0.9, t -test). Results are shown as means±s.e.m. Full size image Increases in glycine site occupancy augment NMDAR responses If the NMDAR glycine site’s occupancy in LA neurons is dynamically modulated by endogenous glycine, released and locally accumulated in quantities corresponding to the level of neuronal activity [8] , then increasing the intensity of presynaptic stimulation should, in principle, decrease the potentiating effect of exogenously applied glycine on evoked NMDAR EPSCs. This is because an increased occupation of the NMDAR glycine site by endogenously released coagonist during stronger presynaptic activation, resulting in recruitment of an increased number of closely localized synaptic inputs, would occlude the effect of NMDAR coagonist added to the external medium. To test this possibility, we first recorded EPSCs at −70 mV and then at +40 mV in each individual neuron in control solution. We then repeated the recordings at both holding potentials in the presence of a saturating concentration of glycine (10 μM), and calculated the NMDA/AMPA ratio for the thalamo-LA EPSCs before (R control ) and after (R coagonist ) the addition of glycine. Importantly, glycine in the concentration used had no effect on the amplitude of AMPAR EPSCs (see Supplementary Fig. S1 ). Indeed, we found that the potentiating effect of glycine on the NMDAR-mediated component of the evoked EPSC, expressed as ratio glycine /ratio control , was negatively correlated with the size of synaptic input ( Fig. 3a–c ; r =−0.58, P <0.01). Thus, exogenous glycine produced less or no potentiation of the larger NMDAR-mediated synaptic currents induced by ‘strong’ presynaptic stimuli (the stimulus intensity was adjusted to produce responses with peak amplitudes >100 pA at −70 mV; Fig. 3c ), while smaller synaptic responses induced by ‘weak’ stimuli (producing EPSCs <100 pA at −70 mV) were enlarged, indicating that activity-dependent coagonist release may modulate the level of NMDAR activation in LA neurons. Thus, the increases in the level of synaptic activation may be translated into augmented NMDAR-mediated synaptic currents. Essentially identical results were obtained when analogous experiments were performed with D- serine, which is transported by astroglia less efficiently ( Fig. 3d–f ; r =−0.5, P =0.028), suggesting that interference from glial glycine transporters [6] in the experiments where exogenous glycine was applied does not explain the results. 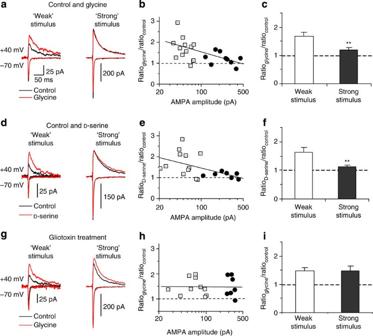Figure 3: Activation of the NMDAR glycine site depends on synaptic strength and requires functional astrocytes. (a) Averaged EPSCs (15 traces) evoked by ‘weak’ stimulation (evoking responses at −70 mV with the amplitude <100 pA) or by ‘strong’ stimulation (amplitude >100 pA) in control solution (black) or in presence of 10 μM glycine (red) in thalamic input at −70 mV (bottom) or +40 mV (top). (b) Magnitude of potentiation of the NMDAR current at +40 mV (measured 40 ms after the peak at −70 mV) by glycine is expressed as the ratioglycine/ratiocontroland plotted as a function of the AMPAR current amplitude at −70 mV. To obtain ratioglycine/ratiocontrol, we calculated the NMDA/AMPA amplitude ratio for the EPSCs before (Rcontrol) and after (Rglycine) addition of a saturating glycine concentration. Potentiating effect of glycine on the ratioglycine/ratiocontrolof evoked EPSCs negatively correlated with the size of synaptic input (n=21 neurons,r=−0.58,P=0.004). (c) Summary plot of the ratioglycine/ratiocontrolat different levels of synaptic activation (‘weak’ stimulus,n=12 neurons; ‘strong’ stimulus,n=9 neurons; **P=0.009 between groups,t-test). (d)D-serine (10 μM) was applied instead of glycine. (e) Ratioglycine/ratiocontrolas a function of the AMPAR current amplitude (n=19 neurons,r=−0.5,P=0.028). (f) Summary plot for experiments indande(‘weak’ stimulus,n=12 neurons; ‘strong’ stimulus,n=7; **P=0.007 between groups,t-test). (g) Slices were pretreated with gliotoxin,L-α-aminoadipic acid (1 mM, ≥90 min). Traces are averaged EPSCs evoked by ‘weak’ stimulation or by ‘strong’ stimulation in control solution (black) or in the presence of 10 μM glycine (red). (h) Ratioglycine/ratiocontrolas a function of the AMPAR current amplitude at −70 mV. Correlation between the effect of glycine on the ratioglycine/ratiocontroland the size of synaptic input was abolished (n=17,r=−0.018,P=0.94). (i) Summary plot for experiments ingandhshowing ratioglycine/ratiocontrol(‘weak’ stimulus,n=10 neurons; ‘strong’ stimulus,n=7,P=0.91 between groups,t-test). Error bars are s.e.m. Figure 3: Activation of the NMDAR glycine site depends on synaptic strength and requires functional astrocytes. ( a ) Averaged EPSCs (15 traces) evoked by ‘weak’ stimulation (evoking responses at −70 mV with the amplitude <100 pA) or by ‘strong’ stimulation (amplitude >100 pA) in control solution (black) or in presence of 10 μM glycine (red) in thalamic input at −70 mV (bottom) or +40 mV (top). ( b ) Magnitude of potentiation of the NMDAR current at +40 mV (measured 40 ms after the peak at −70 mV) by glycine is expressed as the ratio glycine /ratio control and plotted as a function of the AMPAR current amplitude at −70 mV. To obtain ratio glycine /ratio control , we calculated the NMDA/AMPA amplitude ratio for the EPSCs before (R control ) and after (R glycine ) addition of a saturating glycine concentration. Potentiating effect of glycine on the ratio glycine /ratio control of evoked EPSCs negatively correlated with the size of synaptic input ( n =21 neurons, r =−0.58, P =0.004). ( c ) Summary plot of the ratio glycine /ratio control at different levels of synaptic activation (‘weak’ stimulus, n =12 neurons; ‘strong’ stimulus, n =9 neurons; ** P =0.009 between groups, t -test). ( d ) D- serine (10 μM) was applied instead of glycine. ( e ) Ratio glycine /ratio control as a function of the AMPAR current amplitude ( n =19 neurons, r =−0.5, P =0.028). ( f ) Summary plot for experiments in d and e (‘weak’ stimulus, n =12 neurons; ‘strong’ stimulus, n =7; ** P =0.007 between groups, t -test). ( g ) Slices were pretreated with gliotoxin, L- α-aminoadipic acid (1 mM, ≥90 min). Traces are averaged EPSCs evoked by ‘weak’ stimulation or by ‘strong’ stimulation in control solution (black) or in the presence of 10 μM glycine (red). ( h ) Ratio glycine /ratio control as a function of the AMPAR current amplitude at −70 mV. Correlation between the effect of glycine on the ratio glycine /ratio control and the size of synaptic input was abolished ( n =17, r =−0.018, P =0.94). ( i ) Summary plot for experiments in g and h showing ratio glycine /ratio control (‘weak’ stimulus, n =10 neurons; ‘strong’ stimulus, n =7, P =0.91 between groups, t -test). Error bars are s.e.m. Full size image If our model, based on the above-described experiments, is correct, then GO would be expected to have little effect on small intensity evoked EPSCs. We tested this prediction by assaying the effects of enzymatic treatments on EPSCs evoked with minimal stimulation [34] , [35] , [36] . To isolate unitary events, we first selected the recordings where the mean EPSC amplitude showed an all-or-none threshold as a function of stimulation intensity. Second, the unchanged potency (the mean size of responses excluding synaptic failures) of a second response during paired-pulse presynaptic stimulation with a 50-ms interpulse interval was taken as evidence that a single presynaptic fibre was activated ( Fig. 4a ). We found that the amplitude of the NMDAR-mediated component of EPSCs, evoked with minimal stimulation and measured at +40 mV, was sensitive to the treatment with DAAO but not with GO ( Fig. 4c ). This provides further support to the notion that D- serine might be a glycine site agonist at low activity levels, whereas higher degrees of synaptic activation may lead to activity-dependent glycine release, thus resulting in upregulation of NMDAR-mediated synaptic responses through the increases in the glycine site occupancy. 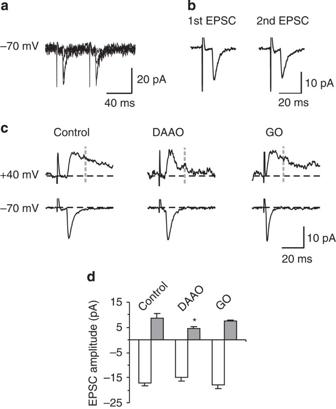Figure 4: NMDAR-mediated component of unitary EPSCs at thalamo-LA synapses is sensitive to DAAO treatment. (a) Superimposed successive EPSCs recorded at −70 mV in response to paired minimal stimulation (50-ms interval). (b) Traces represent average of successes only (potency) for first and second EPSCs. Unchanged potency during paired stimulation at −70 mV was taken as evidence that a single presynaptic fibre was activated34. (c) Left, EPSCs (average traces are shown, 100 events) were evoked in LA neurons with minimal stimulation and recorded at holding potentials of −70 mV (bottom) or +40 mV (top) under control conditions. Middle, recordings were performed following the treatment of slices with DAAO. Right, slices were treated with GO. (d) Summary plot showing the peak amplitude of AMPAR EPSC at −70 mV and the NMDAR-mediated component of the EPSC at +40 mV (dashed lines inc). Control,n=5 neurons; DAAO,n=5; GO,n=6. Amplitude of NMDAR current was decreased following the treatment with DAAO (t-test, *P<0.05 versus control), but it remained unchanged after the treatment with GO (t-test,P=0.2 versus control). Results are shown as means±s.e.m. Figure 4: NMDAR-mediated component of unitary EPSCs at thalamo-LA synapses is sensitive to DAAO treatment. ( a ) Superimposed successive EPSCs recorded at −70 mV in response to paired minimal stimulation (50-ms interval). ( b ) Traces represent average of successes only (potency) for first and second EPSCs. Unchanged potency during paired stimulation at −70 mV was taken as evidence that a single presynaptic fibre was activated [34] . ( c ) Left, EPSCs (average traces are shown, 100 events) were evoked in LA neurons with minimal stimulation and recorded at holding potentials of −70 mV (bottom) or +40 mV (top) under control conditions. Middle, recordings were performed following the treatment of slices with DAAO. Right, slices were treated with GO. ( d ) Summary plot showing the peak amplitude of AMPAR EPSC at −70 mV and the NMDAR-mediated component of the EPSC at +40 mV (dashed lines in c ). Control, n =5 neurons; DAAO, n =5; GO, n =6. Amplitude of NMDAR current was decreased following the treatment with DAAO ( t -test, * P <0.05 versus control), but it remained unchanged after the treatment with GO ( t -test, P =0.2 versus control). Results are shown as means±s.e.m. Full size image Role of astrocytes in modulation of NMDAR function in LA To explore whether astroglia are the source of the NMDAR coagonist released in the course of synaptic activation, as suggested in previous studies at other synapses [8] , [10] , [11] , [12] , we functionally inactivated astrocytes by pretreating slices of the amygdala with external solution containing the gliotoxin, L- α-aminoadipic acid [45] (1 mM). L- α-aminoadipate is known to selectively ablate astrocytes without affecting neuronal functions [46] . Consistent with previous reports, the treatment of slices with gliotoxin in our experiments did not alter the excitability or membrane properties (membrane potential and input resistance) of LA neurons ( Supplementary Fig. S8 ). The efficacy of the AMPAR-mediated neurotransmission at the studied LA synapses, assayed with both input–output curves and paired-pulse ratios also was unaffected by the treatment ( Supplementary Fig. S8 ). In agreement with earlier studies [45] , the treatment caused, however, a nearly twofold increase in the mean area of astrocytic nuclei (glial fibrillary acidic protein (GFAP)-positive cells; Fig. 5a ). 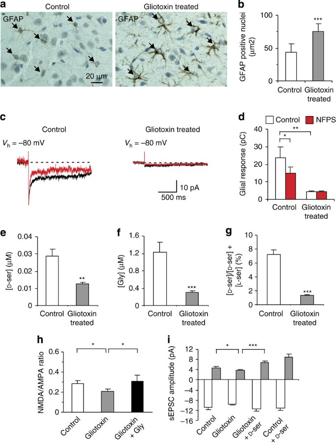Figure 5: Treatment of slices with gliotoxin results in functional inactivation of astrocytes. (a) GFAP-positive cells in LA under control conditions and after gliotoxin treatment. Hypertrophy of GFAP-positive astrocytes was observed in treated slices. Arrows point to individual astrocytes. (b) Gliotoxin treatment led to nuclear swelling in GFAP-positive cells. Graph shows averaged areas of GFAP-positive cell nuclei under control conditions (n=90 cells from three slices) and after gliotoxin treatment (n=108 cells from three treated slices). Data are means±s.d. ***P<0.001 for control versus gliotoxin,t-test. (c) Synaptic responses (averages of 10 traces) were elicited in astrocytes by stimulation of thalamic input before (black trace) and after (red trace) addition of GlyT1 inhibitor NFPS (5 μM) under control conditions and after gliotoxin treatment. (d) Summary of NFPS effects on synaptic charge transfer (picocoulombs, pC) (control,n=6 cells; gliotoxin treatment,n=7 cells). Gliotoxin treatment decreased the amplitude of evoked responses in astrocytes (**P=0.007,t-test). NFPS reduced responses under control conditions (*P=0.03 for control versus NFPS) but had no effect in gliotoxin-treated slices (P=0.7 for control versus NFPS). (e) HPLC analysis. Gliotoxin treatment decreasedD-serine concentration in the perfusate (t-test, **P<0.01). (f) Glycine concentration was also decreased (***P<0.001). (g) Ratio of [D-ser]/[D-ser]+[L-ser] under control conditions and after gliotoxin treatment (***P<0.001). Control data in (e–g) are same as inSupplementary Fig. S2. (h) Evoked NMDAR EPSCs were decreased following gliotoxin treatment. EPSCs were evoked by ‘strong’ stimuli (EPSCs >100 pA at −70 mV). Control,n=25 neurons; gliotoxin,n=16, *P=0.03 versus control; gliotoxin+glycine,n=7, *P=0.02 versus gliotoxin, butP=0.8 versus control. (i) Gliotoxin treatment reduced NMDAR sEPSCs at +40 mV (filled bars). Control,n=15 neurons; gliotoxin,n=20,t-test, *P=0.03 for control versus gliotoxin; gliotoxin+D-serine,n=8, ***P<0.001 versus gliotoxin alone; control+D-serine,n=10,P=0.16 versus gliotoxin+D-serine. Error bars are s.e.m. Figure 5: Treatment of slices with gliotoxin results in functional inactivation of astrocytes. ( a ) GFAP-positive cells in LA under control conditions and after gliotoxin treatment. Hypertrophy of GFAP-positive astrocytes was observed in treated slices. Arrows point to individual astrocytes. ( b ) Gliotoxin treatment led to nuclear swelling in GFAP-positive cells. Graph shows averaged areas of GFAP-positive cell nuclei under control conditions ( n =90 cells from three slices) and after gliotoxin treatment ( n =108 cells from three treated slices). Data are means±s.d. *** P <0.001 for control versus gliotoxin, t -test. ( c ) Synaptic responses (averages of 10 traces) were elicited in astrocytes by stimulation of thalamic input before (black trace) and after (red trace) addition of GlyT1 inhibitor NFPS (5 μM) under control conditions and after gliotoxin treatment. ( d ) Summary of NFPS effects on synaptic charge transfer (picocoulombs, pC) (control, n =6 cells; gliotoxin treatment, n =7 cells). Gliotoxin treatment decreased the amplitude of evoked responses in astrocytes (** P =0.007, t -test). NFPS reduced responses under control conditions (* P =0.03 for control versus NFPS) but had no effect in gliotoxin-treated slices ( P =0.7 for control versus NFPS). ( e ) HPLC analysis. Gliotoxin treatment decreased D- serine concentration in the perfusate ( t -test, ** P <0.01). ( f ) Glycine concentration was also decreased (*** P <0.001). ( g ) Ratio of [ D- ser]/[ D- ser]+[ L- ser] under control conditions and after gliotoxin treatment (*** P <0.001). Control data in ( e – g ) are same as in Supplementary Fig. S2 . ( h ) Evoked NMDAR EPSCs were decreased following gliotoxin treatment. EPSCs were evoked by ‘strong’ stimuli (EPSCs >100 pA at −70 mV). Control, n =25 neurons; gliotoxin, n =16, * P =0.03 versus control; gliotoxin+glycine, n =7, * P =0.02 versus gliotoxin, but P =0.8 versus control. ( i ) Gliotoxin treatment reduced NMDAR sEPSCs at +40 mV (filled bars). Control, n =15 neurons; gliotoxin, n =20, t -test, * P =0.03 for control versus gliotoxin; gliotoxin+ D- serine, n =8, *** P <0.001 versus gliotoxin alone; control+ D- serine, n =10, P =0.16 versus gliotoxin+ D- serine. Error bars are s.e.m. Full size image To provide evidence that the treatment of slices with gliotoxin inactivated astrocytes functionally, we performed electrophysiological recordings from LA astrocytes in control and gliotoxin-treated slices. Astrocytes were identified based on several functional criteria, including very low input resistance (~20 MΩ), more negative membrane potential compared with neurons (>negative than −75 mV), lack of Na + currents during depolarizing voltage steps, and typical linear current–voltage plots (as in [47] ; Supplementary Fig. S9 ). We elicited responses in recorded astrocytes by applying electrical pulses to thalamic input to the LA under control conditions first, and then after the addition of GlyT1 inhibitor N [3-(4′-fluorophenyl)-3-(4′-phenylphenoxy)-propyl]sarcosine (NFPS; 5 μM). The NFPS-sensitive current component, observed in the course of these recordings ( Fig. 5c ; Supplementary Fig. S9 ), was likely reflecting the glycine transporter current through the membrane of a recorded astroglial cell induced by presynaptic stimulation. Interestingly, the NMDAR-mediated component of sEPSCs, measured at +40 mV, was enhanced following the treatment of slices with NFPS, whereas the amplitude of AMPAR sEPSCs at −70 mV remained unchanged ( Supplementary Fig. S10 ). The observed potentiation of single quantum NMDAR responses during GlyT1 blockade likely reflected the fact that spontaneous firing of action potentials has not been prevented in these experiments, as recordings were performed without TTX in the external solution. In the absence of the active uptake, glycine could accumulate in slices, thus resulting in potentiation of NMDAR mEPSCs. We found that the NFPS-sensitive transporter current has been abolished after the treatment of slices with gliotoxin ( Fig. 5c ), providing evidence that astrocytes were functionally inactivated by gliotoxin. We also assayed the effect of gliotoxin (1 mM, 90 min) on levels of D- serine or glycine in the perfusing solution with HPLC analysis, as we did after DAAO or GO treatments. Similar to the experiments with enzymatic treatments, the exposure of slices to gliotoxin-containing solution resulted in significant decreases of extracellular glycine and D- serine concentrations ( Fig. 5e–g ), indicating that gliotoxin treatment was diminishing coagonist concentration under our experimental conditions. Functional inactivation of astrocytes resulted in decreased amplitude of the NMDAR-mediated component of evoked thalamo-LA EPSCs ( Fig. 5h ). Moreover, in the absence of functional astroglia the inverse correlation between the magnitude of potentiation of evoked NMDAR EPSCs by exogenous glycine and the size of synaptic input was no longer observed ( Fig. 3g ; r =−0.018, P =0.94). Under these conditions, exogenous glycine produced similar potentiation of evoked NMDAR EPSCs induced by either ‘weak’ (EPSCs <100 pA at −70 mV) or ‘strong’ (EPSCs >100 pA at −70 mV) presynaptic stimuli ( Fig. 3i ; P <0.005 and P <0.01, respectively). These findings support the notion that glycine, released in the course of evoked synaptic transmission at inputs to the LA (as shown in Fig. 1g ), is likely to originate from astrocytes. Strikingly, inactivation of astrocytes with gliotoxin had an effect on the size of the NMDAR-mediated sEPSCs as well ( Fig. 5i ). Taken together with our HPLC analysis data, the latter finding suggests that ambient D- serine, which enables tonic activation of NMDARs in the absence of evoked synaptic activity ( Fig. 1a ), might be also in part originating from astrocytes. Exogenously applied glycine or D- serine retained the ability to potentiate the NMDAR-mediated component of synaptic responses ( Fig. 5h ), confirming that the function of NMDA receptors was not directly affected by the treatment. Contributions to the induction of LTP in LA What are the implications of these findings for mechanisms of synaptic plasticity in the LA? To differentiate between the functional roles of glycine and D- serine, we explored their contribution in the induction of LTP in slices of the amygdala treated with GO or DAAO, respectively. The amplitude of baseline EPSCs at −70 mV in LTP experiments was kept in a range of 40–60 pA, where the NMDAR glycine site is not saturated by endogenous coagonist in response to presynaptic stimulation ( Fig. 3 ). We found that whereas LTP could be observed in thalamic input to the LA in the DAAO-treated slices ( Figs 6a–c ; P =0.02 versus pre-LTP baseline), the treatment of slices with GO resulted in a complete block of LTP at the same pathway ( Fig. 6e ; P =0.73 versus pre-LTP baseline; P <0.01 versus control LTP). Notably, the magnitude of LTP in DAAO-treated slices was significantly smaller than in control slices ( Fig. 6b ; t -test, P <0.05). The deficits in LTP, observed after enzymatic treatments, were abolished by the addition of D- serine ( Fig. 6d ) or glycine ( Fig. 6f ), respectively. Furthermore, consistent with the role of D- serine in the induction of LTP at thalamo-LA synapses, we found that LTP was suppressed in slices from SR −/− mice when the intensity of presynaptic stimulation was relatively weak (triggering EPSCs with the amplitude ~40–60 pA) ( Fig. 7a ). The NMDAR glycine site is far from being saturated by endogenous coagonist with such stimulation intensities ( Fig. 3 ). However, normal LTP could be observed in slices from SR −/− mice with ‘strong’ presynaptic stimuli, resulting in baseline EPSCs >100–150 pA ( Fig. 7b ). The NMDAR glycine site might be fully occupied by released glycine under these stimulation conditions ( Fig. 3 ), thus overcoming the deficits related to the lack of D- serine production. Consistent with this notion, pretreatment of slices from SR −/− mice with GO suppressed LTP induced with strong presynaptic stimuli ( Fig. 7c ). Overall, these results may suggest a role for both glycine and D- serine in the induction of LTP in the LA. 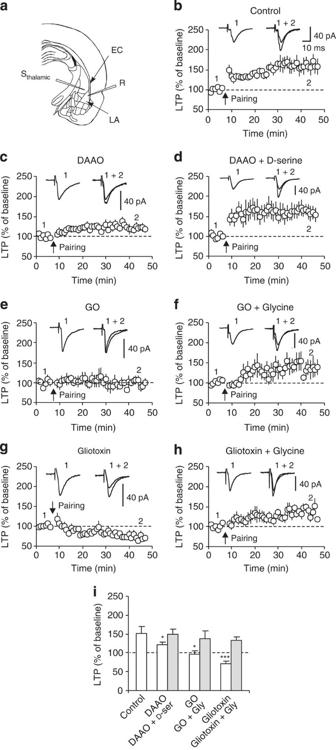Figure 6: Endogenously released glycine andD-serine are required for the induction of LTP at thalamo-LA synapses. (a) Positions of the stimulation (Sthalamic) and recording (R) electrodes. EC, external capsule. (b) LTP of the thalamo-LA EPSC recorded in LA neurons in control external solution (n=10 neurons;P<0.001 versus baseline). Insets show the average of 10 EPSCs recorded before (1), and after (2), the induction (arrow). EPSCs were recorded at a holding potential of −70 mV. Stimulation intensity in LTP experiments was adjusted to produce the baseline EPSCs with amplitude ~40–60 pA. (c) LTP of the thalamo-LA EPSC in DAAO-treated slices (45 min, 0.17 unit ml−1;n=14 neurons,P=0.02 versus baseline). LTP was diminished compared with control LTP shown inb(35 min after the induction,t-test,P<0.05 between groups). (d) LTP in DAAO-treated slices was rescued in the presence of 10 μMD-serine (n=11 neurons,P=0.02 versus baseline). (e) LTP in GO-treated slices was blocked (45 min, 0.04 unit ml−1;n=7 neurons,P=0.73 versus baseline). (f) LTP in GO-treated slices was rescued in the presence of 10 μM glycine (n=8 neurons,P=0.033 versus baseline). (g) LTP was not induced in gliotoxin-treated slices (L-α-aminoadipic acid, 1 mM, ≥90 min) in control solution (n=8 neurons,P<0.001 versus control LTP). (h) LTP in gliotoxin-treated slices was induced in the presence of 10 μM glycine (n=7 neurons,P<0.05 versus baseline). (i) Summary of LTP experiments. *P<0.05 and ***P<0.001 versus control. Results are shown as means±s.e.m. Figure 6: Endogenously released glycine and D- serine are required for the induction of LTP at thalamo-LA synapses. ( a ) Positions of the stimulation (S thalamic ) and recording (R) electrodes. EC, external capsule. ( b ) LTP of the thalamo-LA EPSC recorded in LA neurons in control external solution ( n =10 neurons; P <0.001 versus baseline). Insets show the average of 10 EPSCs recorded before (1), and after (2), the induction (arrow). EPSCs were recorded at a holding potential of −70 mV. Stimulation intensity in LTP experiments was adjusted to produce the baseline EPSCs with amplitude ~40–60 pA. ( c ) LTP of the thalamo-LA EPSC in DAAO-treated slices (45 min, 0.17 unit ml −1 ; n =14 neurons, P =0.02 versus baseline). LTP was diminished compared with control LTP shown in b (35 min after the induction, t -test, P <0.05 between groups). ( d ) LTP in DAAO-treated slices was rescued in the presence of 10 μM D- serine ( n =11 neurons, P =0.02 versus baseline). ( e ) LTP in GO-treated slices was blocked (45 min, 0.04 unit ml −1 ; n =7 neurons, P =0.73 versus baseline). ( f ) LTP in GO-treated slices was rescued in the presence of 10 μM glycine ( n =8 neurons, P =0.033 versus baseline). ( g ) LTP was not induced in gliotoxin-treated slices ( L- α-aminoadipic acid, 1 mM, ≥90 min) in control solution ( n =8 neurons, P <0.001 versus control LTP). ( h ) LTP in gliotoxin-treated slices was induced in the presence of 10 μM glycine ( n =7 neurons, P <0.05 versus baseline). ( i ) Summary of LTP experiments. * P <0.05 and *** P <0.001 versus control. Results are shown as means±s.e.m. 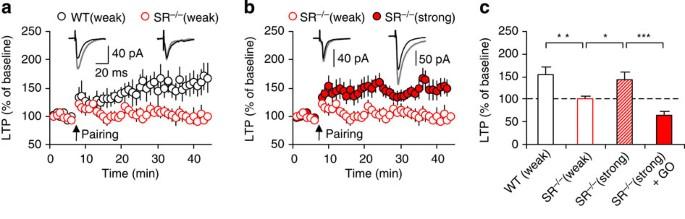Figure 7: LTP in slices from SR−/−and control littermate mice. (a) LTP of the thalamo-LA EPSC recorded in LA neuron in slices from control (black) and SR−/−mice (red) (data from seven control mice,n=9 neurons,P<0.02 versus baseline; and from seven SR−/−mice,n=9 neurons,P=0.4 versus baseline). Insets show the average of 10 EPSCs recorded before and 35 min after LTP induction (at arrow). The EPSCs were recorded at a holding potential of −70 mV. To induce LTP, postsynaptic depolarization to +40 mV was paired with 80 presynaptic stimuli at a frequency of 2 Hz. The intensity of stimulation was adjusted to produce baseline EPSCs with the amplitude ~40–60 pA (‘weak’ stimulation). (b) Similar toabut the intensity of stimulation was adjusted to produce baseline EPSCs with the amplitude >100–150 pA (‘strong’ stimulation; filled red symbols; data from six SR−/−mice,n=8 neurons,P<0.01 versus baseline). The graph showing a lack of LTP in SR−/−mice with ‘weak’ presynaptic stimuli is the same as ina. (c) Summary of LTP results. Control mice (weak stimulation),n=9 neurons from seven mice; SR−/−mice (weak stimulation),n=9 neurons from seven mice,t-test, **P<0.01 between groups). LTP was rescued in slices from SR−/−mice when baseline responses were induced by stronger stimuli,n=8 neurons from six mice;t-test, *P<0.05 versus LTP in SR−/−mice with weak stimulation. LTP in larger inputs in slices from SR−/−mice is suppressed in GO-treated slices,n=8 neurons from four SR−/−mice,t-test, ***P<0.001 versus SR−/−(strong). Results are shown as means±s.e.m. Full size image Figure 7: LTP in slices from SR −/− and control littermate mice. ( a ) LTP of the thalamo-LA EPSC recorded in LA neuron in slices from control (black) and SR −/− mice (red) (data from seven control mice, n =9 neurons, P <0.02 versus baseline; and from seven SR −/− mice, n =9 neurons, P =0.4 versus baseline). Insets show the average of 10 EPSCs recorded before and 35 min after LTP induction (at arrow). The EPSCs were recorded at a holding potential of −70 mV. To induce LTP, postsynaptic depolarization to +40 mV was paired with 80 presynaptic stimuli at a frequency of 2 Hz. The intensity of stimulation was adjusted to produce baseline EPSCs with the amplitude ~40–60 pA (‘weak’ stimulation). ( b ) Similar to a but the intensity of stimulation was adjusted to produce baseline EPSCs with the amplitude >100–150 pA (‘strong’ stimulation; filled red symbols; data from six SR −/− mice, n =8 neurons, P <0.01 versus baseline). The graph showing a lack of LTP in SR −/− mice with ‘weak’ presynaptic stimuli is the same as in a . ( c ) Summary of LTP results. Control mice (weak stimulation), n =9 neurons from seven mice; SR −/− mice (weak stimulation), n =9 neurons from seven mice, t -test, ** P <0.01 between groups). LTP was rescued in slices from SR −/− mice when baseline responses were induced by stronger stimuli, n =8 neurons from six mice; t -test, * P <0.05 versus LTP in SR −/− mice with weak stimulation. LTP in larger inputs in slices from SR −/− mice is suppressed in GO-treated slices, n =8 neurons from four SR −/− mice, t -test, *** P <0.001 versus SR −/− (strong). Results are shown as means±s.e.m. Full size image Inactivation of astrocytes, which are required for the activity-dependent glycine release in the LA ( Fig. 3g–i ), with L- α-aminoadipic acid not only prevented the induction of LTP in thalamic input ( Fig. 6g ; P <0.001 versus control LTP) but resulted in depression of synaptic transmission. Similar depression of synaptic responses was reported previously at CA1 hippocampal synapses in response to LTP-inducing stimulation in slices that were treated with a different gliotoxin, fluoroacetate [12] . Gliotoxin effect on LTP was reversed by the addition of glycine to the external solution ( Fig. 6h , providing evidence that LTP deficits were not due to the effect of gliotoxin on slice viability. As demonstrated previously, the magnitude of NMDAR-dependent LTP at central synapses is determined by the degree of NMDAR activation during the induction process [48] . To explore whether NMDAR function is affected by the activity-dependent release of the glycine site agonist during the induction of LTP at LA synapses, we determined the total synaptic charge transfer (Qsum) during the delivery of LTP-inducing stimulation, summarizing all 80 EPSCs in the train at +40 mV, under different experimental conditions ( Fig. 8a–c ). The Qsum +40 mV values for the EPSCs composed of both AMPAR- and NMDAR-mediated components were then normalized by the averaged charge transfer during baseline AMPAR EPSCs at −70 mV (Qmean −70 mV ). Consistent with a role of activity-dependent glycine release in maintaining the necessary level of NMDAR activation in the course of LTP induction, we found that the treatment of slices with GO or L- α-aminoadipic acid resulted in a decreased Qsum +40 mV /Qmean −70 mV ratio, reflecting a decreased level of NMDAR activation. The addition of D- serine or glycine to the external solution led to increases in the Qsum +40 mV /Qmean −70 mV ratio in slices treated with DAAO or GO, respectively ( Fig. 8b ), and enhanced potentiation, indicating that the machinery of LTP remained intact following the enzymatic treatment of slices. As expected, the magnitude of LTP positively correlated with the Qsum +40 mV /Qmean −70 mV values during LTP-inducing stimulation ( r =0.92; P =0.009; Fig. 8c ), showing that the level of NMDAR activation at LA synapses during the induction process determines the inducibility of LTP. Together, these findings show that release of glycine, in quantities corresponding to presynaptic activity levels, and tonically present D- serine are necessary for the induction of LTP at thalamo-amygdala synapses. 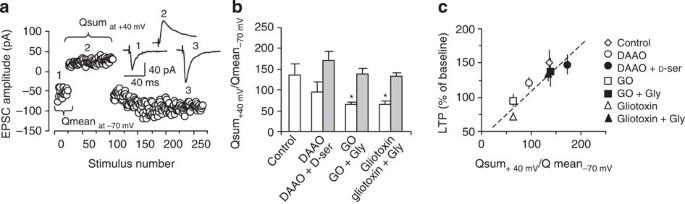Figure 8: Endogenous glycine andD-serine maintain the required level of NMDAR activation in the course of LTP induction. (a) LTP of the thalamo-LA EPSC. Insets show averaged EPSCs recorded before (1), during (2) and after (3) the induction of LTP. The EPSCs were recorded at −70 mV in (1) and (3), or at +40 mV in (3). The EPSC peak amplitudes at −70 mV before and after the induction of LTP and the amplitudes measured 40 ms after the peak at +40 mV during the induction are plotted as a function of stimulus number. Brackets show the periods where Qmean−70 mVand Qsum+40 mVvalues in the course of the experiment were calculated. (b) The values of Qsum+40 mV/Qmean−70 mVratio during the induction of LTP at different experimental conditions. Qsum is the total synaptic charge transfer at +40 mV during LTP induction, summarizing all 80 EPSCs. The values of Qsum were normalized by the averaged charge transfer during baseline AMPAR EPSCs at −70 mV (Qmean−70 mV). Control,n=10 neurons; DAAO treatment,n=14; DAAO+D-serine,n=11; *P=0.03 versus DAAO group; GO treatment,n=7; *P=0.018 versus control; GO+glycine,n=8,P<0.001 versus GO group; gliotoxin treatment (L-α-aminoadipic acid, 1 mM, ≥90 min),n=8,P=0.022 versus control; glycine after gliotoxin treatment,n=7,P<0.001 versus gliotoxin treatment. (c) The magnitude of LTP is positively correlated with the Qsum+40mV/Qmean−70mVvalues during the induction (r=0.91;P<0.01). Results are shown as means±s.e.m. Figure 8: Endogenous glycine and D- serine maintain the required level of NMDAR activation in the course of LTP induction. ( a ) LTP of the thalamo-LA EPSC. Insets show averaged EPSCs recorded before (1), during (2) and after (3) the induction of LTP. The EPSCs were recorded at −70 mV in (1) and (3), or at +40 mV in (3). The EPSC peak amplitudes at −70 mV before and after the induction of LTP and the amplitudes measured 40 ms after the peak at +40 mV during the induction are plotted as a function of stimulus number. Brackets show the periods where Qmean −70 mV and Qsum +40 mV values in the course of the experiment were calculated. ( b ) The values of Qsum +40 mV /Qmean −70 mV ratio during the induction of LTP at different experimental conditions. Qsum is the total synaptic charge transfer at +40 mV during LTP induction, summarizing all 80 EPSCs. The values of Qsum were normalized by the averaged charge transfer during baseline AMPAR EPSCs at −70 mV (Qmean −70 mV ). Control, n =10 neurons; DAAO treatment, n =14; DAAO+ D- serine, n =11; * P =0.03 versus DAAO group; GO treatment, n =7; * P =0.018 versus control; GO+glycine, n =8, P <0.001 versus GO group; gliotoxin treatment ( L- α-aminoadipic acid, 1 mM, ≥90 min), n =8, P =0.022 versus control; glycine after gliotoxin treatment, n =7, P <0.001 versus gliotoxin treatment. ( c ) The magnitude of LTP is positively correlated with the Qsum +40 mV /Qmean −70 mV values during the induction ( r =0.91; P <0.01). Results are shown as means±s.e.m. Full size image Our results provide evidence that both glycine and D- serine serve as endogenous NMDAR glycine site agonists in the LA, but the identity of the agonist might be determined by synaptic activity levels. Ambient D- serine may maintain activation of NMDARs in LA neurons in the absence of evoked synaptic events, while activity-dependent release of glycine from astrocytes is implicated in activation of NMDARs during afferent stimulation. Although supporting a role for both endogenous glycine and D- serine [10] , [11] in the induction of LTP, our findings emphasize the contribution of glycine released by activity at stronger synaptic inputs in the induction process. Present study complements the results of an earlier published work where we demonstrated that different spatiotemporal patterns of presynaptic activity could be translated into different levels of NMDAR activation in the hippocampus [8] . As similar synaptic rules are implicated in activity-dependent regulation of NMDARs at synapses in two different regions of the brain, the amygdala and the hippocampus, the described modulation of NMDAR function through activity-dependent changes of the glycine site occupancy might reflect a general regulatory mechanism of NMDAR function. In agreement with our findings, coexistence of two glycine site agonists, glycine and D- serine, has been demonstrated previously at synaptic inputs to retinal ganglion cells [22] . In this earlier study, the glycine site was shown to be saturated by glycine during evoked release, whereas it was far from being saturated under baseline conditions. It appears, however, that the identity of the NMDAR coagonist, glycine or D- serine, might be synapse specific. Thus, it has been shown that D- serine may serve as the endogenous NMDAR coagonist in the course of evoked synaptic transmission in the hypothalamic supraoptic nucleus [11] . The results of another study also suggested that glycine is not an endogenous coagonist of synaptic NMDARs at CA3–CA1 synapses in the hippocampus [38] . This conclusion was based on the outcome of experiments where the treatment of slices with GO did not reduce the amplitude of evoked field potentials. However, AMPA receptors were blocked during these recordings by the selective antagonist. Our previous findings in the hippocampus [8] indicate that activation of AMPA receptors is required for activity-dependent glycine release, thus possibly explaining the lack of GO effect on pharmacologically isolated NMDAR-mediated fEPSPs in the mentioned work [38] . The differences in activity/penetration of the enzymes, DAAO or GO, in situ are an unlikely explanation for our results for the following reasons. Thus, GO and DAAO do not differ in respect to their physicochemical properties, which could possibly affect penetration of the enzymes into the tissue or their activity, including molecular mass, Rossmann fold and cofactors. Moreover, it has been demonstrated previously using HPLC analysis that there are no differences in GO or DAAO activities under comparable conditions in the brain slices [11] . The effects of DAAO or GO were specifically linked to their enzymatic activities, using inactive DAAO [16] or GO variants [38] . Importantly, our experiments with either DAAO or GO, performed under similar conditions, had positive functional controls for each treatment, as DAAO was affecting spontaneous sEPSCs, whereas GO was affecting evoked responses. Therefore, the differences in enzymatic activities or penetration could not explain the differential effects of DAAO or GO on spontaneous versus evoked responses in our study. Our findings suggest an interesting possibility that both ambiently present D- serine, and glycine released by synaptic activity might contribute to the induction of LTP. D- serine may contribute to the induction in smaller synaptic inputs, where the release of glycine alone would be insufficient to reach the level of NMDAR activation required for the induction of LTP. In larger inputs, the deficits in tonic activation of NMDARs could be completely overridden by glycine released in response to presynaptic stimuli in quantities saturating the NMDAR glycine site, and, therefore, the activity-dependent glycine release alone would be sufficient to support the induction of LTP. Consistent with the latter possibility, we found that LTP induced with strong presynaptic stimuli was suppressed following a pretreatment of slices from SR −/− mice with GO. We found previously that modulation of the NMDAR function through local glutamate-induced glycine release is spatially restricted [8] . Therefore, transient increases in activation of NMDARs at neighbouring synapses due to glycine release could mediate input specificity of LTP during associative learning, specifically during the acquisition of fear memory, whereas ambient D- serine would maintain tonic activation of NMDARs, creating conditions for the induction of plasticity forms that are not restricted to specific pathways. Notably, it has been demonstrated recently that genetic manipulations in mice, which result in obliterated G q protein-coupled receptor-induced Ca 2+ signalling in astrocytes, had no effect on LTP in the CA1 area of the hippocampus [17] , thus arguing against the involvement of Ca 2+ -dependent release of gliotransmitters in LTP induction. Unlike D- serine, which might be released by astrocytes via Ca 2+ -dependent exocytosis [16] , the release of glycine does not require astrocytic Ca 2+ fluxes. Glycine, accumulated in astrocytes by the Na + -coupled glycine transporter GlyT1, can be released by reverse transport in response to local increases in the intra-astrocyte Na + concentration resulting from activation of glial AMPA receptors, thus increasing the extracellular concentration of glycine to the micromolar range [14] , [15] , [23] , [49] . In summary, different degrees of the NMDAR glycine binding site occupancy by endogenous glycine at LA synapses result in different levels of the NMDA receptor activation, creating conditions for the activity-dependent upregulation of the NMDAR function, and, therefore, contributing to the mechanisms of synaptic plasticity in auditory CS stimulus pathways, known to underlie the acquisition of CS fear memory [39] . Electrophysiological recordings in brain slices Slices of the amygdala (250–300 μm) were prepared from 3- to 5-week-old Sprague-Dawley rats of either sex or from SR −/− and control (wild-type littermates) mice [43] (both males and females) with a vibratome. Slices were continuously superfused in solution containing (in mM): 119 NaCl, 2.5 KCl, 2.5 CaCl 2 , 1.0 MgSO 4 , 1.25 NaH 2 PO 4 , 26.0 NaHCO 3 , 10 glucose and 0.05 picrotoxin, and equilibrated with 95% O 2 and 5% CO 2 (pH 7.3–7.4) at physiological temperature (35–36 °C). Whole-cell recordings of compound or sEPSCs were obtained from pyramidal neurons in the LA under visual guidance (DIC/infrared optics) with an EPC-10 amplifier and Pulse v8.67 software (HEKA Elektronik). Evoked synaptic responses were triggered by field stimulation of the internal capsule (thalamic input) at 0.1 Hz with a fine-tipped (~2 μm) glass stimulation pipette. The recording patch electrodes (3–6 MΩ resistance) contained (in mM) 120 Cs-methane-sulfonate, 5 NaCl, 1 MgCl 2 , 0.2 EGTA, 10 HEPES, 2 MgATP and 0.1 NaGTP (adjusted to pH 7.2 with CsOH). Currents were filtered at 1 kHz and digitized at 5 kHz. The AMPAR EPSC amplitude was measured at a holding potential of −70 mV as the difference between the mean current during a prestimulus baseline and the mean current over a 1- to 2-ms window at the response peak. The NMDAR-mediated component of the EPSC at +40 mV was measured 40 ms after the peak of the AMPAR ESPCs (recorded at −70 mV) for evoked responses and 15 ms after the peak for sEPSCs or mEPSCs. NMDA/AMPA amplitude ratio was calculated by dividing the amplitude of the NMDAR component measured 40 ms after the peak at +40 mV by the peak AMPA receptor EPSC measured at −70 mV. For induction of LTP, 80 presynaptic stimuli, delivered at 2 Hz to the fibres in thalamic input, were paired with postsynaptic depolarization to +40 mV (ref. 34 ). Summary LTP graphs were constructed by normalizing data in 60 s epochs to the mean value of the baseline EPSCs recorded at a holding potential of −70 mV. mEPSCs were recorded in the presence of 1 μM TTX. Both sEPSCs and mEPSCs were analysed using Mini Analysis Program v6.0.7 (Synaptosoft Inc.). Spontaneous synaptic events were recorded first at −70 mV for ~5 min (to collect 100–150 events, and then at +40 mV in the presence of 50 μM picrotoxin. Data were analysed offline. The area threshold criterion, as well as the fast rise time, was used to detect the spontaneous synaptic events and eliminate the peaks that arise from noise. All animal procedures were approved by McLean Hospital’s Institutional Animal Care and Use Committee. HPLC analysis In these experiments, slices of the amygdala were bathed in the external solution at physiological temperatures (35–36 °C). The samples for HPLC analysis were obtained under four different conditions: control where perfusing solution was in contact with untreated slices; perfusing solution was obtained after the treatment of slices with either GO (0.04 U ml −1 ) or DAAO (0.17 U ml −1 ) for 45 min; solution was obtained after the treatment of slices with gliotoxin ( L- α-aminoadipic acid, 1 mM) for 90 min. Thalamo-LA synapses were infrequently stimulated (at 0.1 Hz) during the treatments. The sample of conditioned medium, retrieved for HPLC analysis after perfusion of control and treated slices, was lyophilized and stored at −80 °C. Each sample was resuspended/dissolved in 1 ml MilliQ water, vortexed for 1 min, bath sonicated for 6 min at room temperature and cleared up by centrifugation at 13,000 r.p.m. and 4 °C for 30 min. Five to ten millilitres of samples were then subjected to pre-column derivatization with o -phthaldialdehyde/ N -acetyl -L- cysteine in borate buffer (0.1 M, pH 10.4) (ref. 50 ). Diastereoisomer derivatives were resolved on a Luna 5μ C18(2) 100A (Phenomenex, 4.6 × 150 mm) reversed phase column in isocratic conditions. The mobile phase consisted in sodium acetate buffer (0.1 M, pH 6.2) added with 1% tetrahydrofuran (0.6 ml min −1 flow rate). After every single run a washing step in 0.1 M sodium acetate buffer, 3% tetrahydrofuran and 47% acetonitrile was performed. Identification and quantification of glycine, and D- and L-isomer of serine was based on retention times and peak areas, compared with those associated with external standards. Standards were prepared as 1 mM stock solution in MilliQ water. Calibration curves were built by injecting increasing amount of standards (0.01–0.5 μM range for D- and L- serine, 0.025–1 μM range for glycine). Immunohistochemistry and quantitative analysis Amygdalar slices (300 μm in thickness) from one side of the brain were incubated in oxygenated artificial cerebrospinal fluid for 90 min as a control, and slices from another side were incubated in oxygenated artificial cerebrospinal fluid containing 1 mM L- 2-aminoadipic acid for 90 min. Then, slices were fixed in 4% paraformaldehyde for 72 h, paraffin-embedded and sectioned into thin slides (5 μm in thickness). After antigen retrieval, slides were incubated with rabbit polyclonal antibody against GFAP (1:2,000; Abcam). Rabbit EnVision was used as a secondary antirabbit antibody (Daco). Antibody binding was visualized with diaminobenzidine as chromogen substrate and counter stained with haematoxylin. Zeiss Axioskop 2 Plus microscope interfaced with the system of Stereo Investigator 6.0 (Microbrightfield Inc., Williston, Vermont) was used for a quantitative analysis. The data for quantitative analysis were obtained from three sections, each from individual gliotoxin-treated slice, and three sections from control slices. The numeric densities for astroglial cells and morphological changes were assessed within the LA. The sampling grid (900 μm 2 of grid size in the total area of 8,100 μm 2 ) was used to select the stained cells. In each sampling grid, the size of soma was manually traced on the GFAP-positive cells under × 40 objective with an assistance of the Stereo Investigator system. The tracings were made at the focal plane in which the cell somas were maximal in size and cell nuclei were clearly visible. Soma sizes were estimated by the area (μm 2 ) measured for individual astroglial cells. In this manner, 23–47 astroglial cell profiles were measured per each section of the LA. How to cite this article: LI, Y. et al . Identity of endogenous NMDAR glycine site agonist in amygdala is determined by synaptic activity level. Nat. Commun. 4:1760 doi: 10.1038/ncomms2779 (2013).